The X-ray crystal structure of the euryarchaeal RNA polymerase in an open-clamp configuration The archaeal transcription apparatus is closely related to the eukaryotic RNA polymerase II (Pol II) system. Archaeal RNA polymerase (RNAP) and Pol II evolved from a common ancestral structure and the euryarchaeal RNAP is the simplest member of the extant archaeal–eukaryotic RNAP family. Here we report the first crystal structure of euryarchaeal RNAP from Thermococcus kodakarensis ( Tko ). This structure reveals that the clamp domain is able to swing away from the main body of RNAP in the presence of the Rpo4/Rpo7 stalk by coordinated movements of these domains. More detailed structure–function analysis of yeast Pol II and Tko RNAP identifies structural additions to Pol II that correspond to the binding sites of Pol II-specific general transcription factors including TFIIF, TFIIH and Mediator. Such comparisons provide a framework for dissecting interactions between RNAP and these factors during formation of the pre-initiation complex. Archaeal proteins associated with genome maintenance and gene expression have extensive functional and structural similarities with their eukaryotic counterparts [1] , [2] . This congruence is especially true for the archaeal transcription machinery, and there is a striking structural similarity between archaeal and eukaryotic RNA polymerases (RNAPs) [3] , [4] , [5] . Comparing the pre-initiation complex (PIC) formation of the archaeal and three eukaryotic transcription systems (Pol I, II and III) revealed that all RNAPs use a core subset of structurally and functionally related transcription factors to initiate promoter-dependent transcription [6] . All factors are auxiliary for the archaeal and Pol II transcription systems; however, some factors are bona fide RNAP subunits for the Pol I and Pol III transcription systems. Archaeal RNAP is most closely related to Pol II in subunit composition, and their requirements for general transcription factors (GTFs) exactly match a subset of GTFs required for the activities of Pol II. Archaeal RNAP requires only two monomeric GTFs—TBP and TFB—for PIC formation and transcription in vitro , although a third monomeric GTF—TFE—can assist PIC formation in vitro and appears essential factor in vivo [1] , [3] , [7] , [8] . PIC formation with Pol II requires a more complex set of GTFs, with minimally six GTFs (TFIIA, TFIIB, TFIID/TBP, TFIIE, TFIIF and TFIIH) and the Mediator complex is also required for promoter-specific transcription [7] , [9] , [10] . Archaea consists of two major phyla, Euryarchaeota and Crenarchaeota, and phylogenetic analyses of the essential components in DNA replication, transcription and translation suggested that Euryarchaeota have retained a set of features that more likely represent the ancestral form present in the last common ancestor of eukaryotes and archaea [11] , [12] . 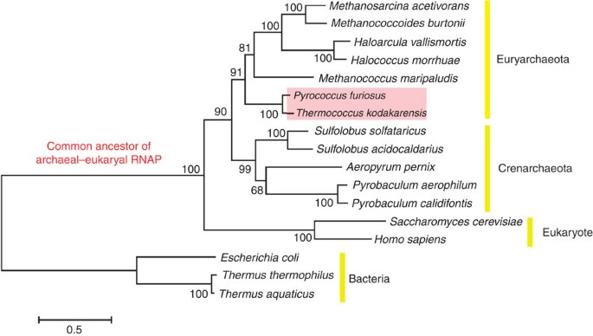Figure 1: Phylogenetic analysis of the largest subunit of RNAP in bacteria, euryarchaeota, crenarchaeota and eukaryotes. Maximum-likelihood phylogenetic tree made with the largest subunit of RNAP (β′ of bacterial RNAP, Rpo1′+Rpo1′′ of archaeal RNAP, and Rpb1 of eukaryotic RNAP II) rooted with bacterial sequences. Bootstrap support based on 500 replicates is shown at each node. Scale bar represents the average number of substitutions per residues. The position of common ancestor of archaeal–eukaryal RNAP is indicated in red. An order ofThermococcalesincludingPfuandTkois highlighted. Euryarchaeal RNAP is composed of 11 subunits and all subunits are conserved in the archaeal–eukaryotic RNAP family ( Supplementary Table 1 ), whereas crenarchaeal RNAP contains two additional subunits Rpo8 and Rpo13 (refs 13 , 14 ). Although structural and functional similarities between archaeal and Pol II transcription machineries have been known for decades, precise comparison of these RNAPs generate new insights about structural motifs of RNAP that participate in the assembly of the PIC and transcription regulation. We report the crystal structure of Thermococcus kodakarensis ( Tko ) RNAP at 3.5 Å resolution, which reveals the molecular details of the open-clamp state of the RNAP in the presence of the Rpo4/Rpo7 stalk. Structure-guided sequence alignment between Tko RNAP and yeast Pol II postulates how retained insertions and modifications to Pol II during RNAP evolution have been utilized to establish interactions with Pol II-specific GTFs and Mediator. Our structure–function analysis provides insight regarding the evolution of multisubunit RNAPs with their binding factors and also serves as a guide for studying the physical interactions between Pol II and transcription regulators. Tko RNAP purification and crystallization The phylogenetic analysis of the largest subunit of cellular RNAPs indicates that among Euryarchaeota, Thermococcales including Tko is the closest forms of RNAP to the common ancestor of the archaeal–eukaryotic RNAP family ( Fig. 1 ). Therefore, Tko RNAP can be used as an ideal reference to analyse the structure and evolution of archaeal–eukaryotic RNAP family [15] . Tko RNAP purified directly from cells contains substoichiometric amounts of TFE [16] , and this heterogeneity likely precluded crystallization attempts. Tko RNAP purified from a Δrpo4 strain yields an enzyme that lacks Rpo4, Rpo7 and TFE [16] . Introduction of recombinant Rpo4 and Rpo7 into this TFE-free RNAP reformed the full 11-subunit enzyme ( Supplementary Fig. 1 ) that could be crystallized successfully. The structure was determined by molecular replacement using the Sulfolobus solfataricus RNAP structure (PDB ID 3HKZ) [1] as a search model. 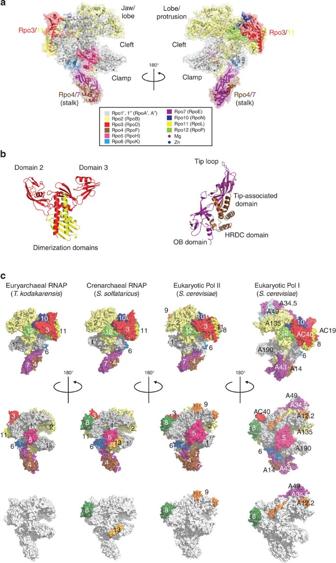Figure 2: Crystal structures of theTkoRNAP and other members of archaeal–eukaryotic RNAP family. (a)TkoRNAP structure in a ribbon model along with a transparent molecular surface. Each subunit is denoted by a unique colour and was labelled. Two sets of nomenclatures, one for traditional (in parenthesis) and the other based on the eukaryotic terminology, are shown. Some structural features are labelled. (b) Crystal structures of Rpo3/Rpo11 (left) and Rpo4/Rpo7 (right) complexes. Domains are labelled. Each subunit is coloured as ina. (c) Surface representations of the archaeal and eukaryotic RNAPs. Each subunit is denoted by a unique colour and labelled. Orthologous subunits are depicted by the same colour. In a bottom panel, common subunits are shown in grey. We also solved the high-resolution structures of heterodimers formed by Tko RNAP subunits including Rpo3/Rpo11 (1.6 Å) and Rpo4/Rpo7 (2.3 Å; Supplementary Table 2 ), and replacement with these structures allowed refinement of the final structure of Tko RNAP at 3.5 Å resolution with high quality ( Supplementary Fig. 2 and Supplementary Table 2 ). Figure 1: Phylogenetic analysis of the largest subunit of RNAP in bacteria, euryarchaeota, crenarchaeota and eukaryotes. Maximum-likelihood phylogenetic tree made with the largest subunit of RNAP (β′ of bacterial RNAP, Rpo1′+Rpo1′′ of archaeal RNAP, and Rpb1 of eukaryotic RNAP II) rooted with bacterial sequences. Bootstrap support based on 500 replicates is shown at each node. Scale bar represents the average number of substitutions per residues. The position of common ancestor of archaeal–eukaryal RNAP is indicated in red. An order of Thermococcales including Pfu and Tko is highlighted. Full size image The Tko RNAP structure The overall shape of Tko RNAP resembles that of the crenarchaeal RNAP and eukaryotic Pol I and Pol II ( Fig. 2 ). All subunits of Tko RNAP are conserved in archaeal–eukaryotic RNAPs supporting that the Tko RNAP structure represents the closest form to their common ancestor ( Fig. 2c ). Superposition of the Tko RNAP structure with the Sso RNAP and yeast Pol II structures, both captured in the closed-clamp conformation [17] , [18] , reveals that the Tko RNAP clamp is in an open state ( Fig. 3a ). In the Tko RNAP structure, the position of DNA-binding clamp (Rpo1′ residues 1–322, Rpo1′′ residues 332–391 and Rpo2 residues 1,058–1,123) is widely opened and hinged away from the main channel. The Tko RNAP structure fits nicely into the cryo-EM map of the closely related Pyrococcus furiosus ( Pfu ) RNAP [19] ( Fig. 1 and Supplementary Table 1 ), with the exception of the DNA-binding clamp ( Fig. 3b ). This difference adumbrates that the archaeal–eukaryotic RNAPs can readily adopt different clamp conformations in solution. The clamp of Tko RNAP swings away from the main channel and undergoes a clockwise rotation of ~21.3° compared with the clamp position in Sso RNAP ( Fig. 3c ). The repositioning of the clamp—termed opening—is coupled with the movement and counterclockwise rotation of Rpo4/Rpo7 stalk of ~12°, which allows the clamp to open without a steric hindrance with the stalk ( Supplementary Movie 1 ). This concerted movement resolves, in molecular detail, two concerns raised from the interpretations of the crystallographic studies of yeast Pol II: (1) the suggestion that the clamp may only be opened in the absence of the stalk, and (2) the suggestion that a tip loop of the stalk binding underneath the clamp may serve as a wedge to restrict clamp opening [17] . The Tko RNAP structure indicates that the clamp opening is possible in the presence of the stalk in archaeal RNAP and likely Pol II ( Fig. 3d ), and there is substantial evidence in support of such from cryo-EM structural studies of Pol II. Pol II alone [20] and Pol II in complex with GTFs [21] were best fitted by a model of Pol II in the open-state clamp configuration, and in each of these studies, the stalk was present. Using the Tko RNAP structure, a model of Pol II showing probable concerted transitions of the clamp and stalk domains was developed, indicating that these domains are able to open without a steric clash ( Supplementary Movie 2 ). Figure 2: Crystal structures of the Tko RNAP and other members of archaeal–eukaryotic RNAP family. ( a ) Tko RNAP structure in a ribbon model along with a transparent molecular surface. Each subunit is denoted by a unique colour and was labelled. Two sets of nomenclatures, one for traditional (in parenthesis) and the other based on the eukaryotic terminology, are shown. Some structural features are labelled. ( b ) Crystal structures of Rpo3/Rpo11 (left) and Rpo4/Rpo7 (right) complexes. Domains are labelled. Each subunit is coloured as in a . ( c ) Surface representations of the archaeal and eukaryotic RNAPs. Each subunit is denoted by a unique colour and labelled. Orthologous subunits are depicted by the same colour. In a bottom panel, common subunits are shown in grey. 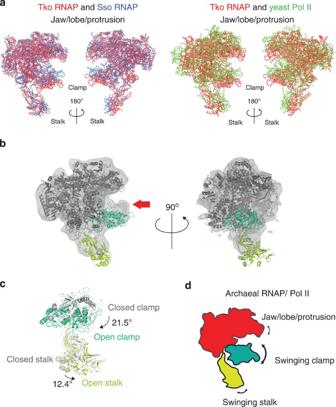Figure 3: Opening and closing of the DNA-binding clamp of RNAP. (a) The structure ofTkoRNAP is superimposed on the structures ofSsoRNAP (left, blue, PDB: 3 HKZ) and yeast Pol II (right, green, PDB: 1 WCM) using the enzyme active sites as references. (b) Cryo-EM density map ofPfuRNAP (light grey mesh, EMD-1711) is overlaid with theTkoRNAP structure (main body of RNAP, grey; clamp, dark cyan; Rpo4/Rpo7 stalk, yellow-green; active site Mg, magenta sphere). The clamp ofPfuRNAP is indicated by a red arrow and in a closed-state. (c) Proposed motions of the clamp and stalk of archaeal RNAP. The open clamp (dark cyan) and stalk (yellow-green) observed in theTkoRNAP structure are superimposed on the closed clamp and stalk (grey) in theSsoRNAP structure. Motions and angles of the clamp and stalk from the closed to the open conformations are indicated. (d) Schematic representation of archaeal RNAP/Pol II showing the mobility of the DNA-binding cleft and the stalk. Full size image Figure 3: Opening and closing of the DNA-binding clamp of RNAP. ( a ) The structure of Tko RNAP is superimposed on the structures of Sso RNAP (left, blue, PDB: 3 HKZ) and yeast Pol II (right, green, PDB: 1 WCM) using the enzyme active sites as references. ( b ) Cryo-EM density map of Pfu RNAP (light grey mesh, EMD-1711) is overlaid with the Tko RNAP structure (main body of RNAP, grey; clamp, dark cyan; Rpo4/Rpo7 stalk, yellow-green; active site Mg, magenta sphere). The clamp of Pfu RNAP is indicated by a red arrow and in a closed-state. ( c ) Proposed motions of the clamp and stalk of archaeal RNAP. The open clamp (dark cyan) and stalk (yellow-green) observed in the Tko RNAP structure are superimposed on the closed clamp and stalk (grey) in the Sso RNAP structure. Motions and angles of the clamp and stalk from the closed to the open conformations are indicated. ( d ) Schematic representation of archaeal RNAP/Pol II showing the mobility of the DNA-binding cleft and the stalk. Full size image In the Pol I crystal structure, the main cleft adopts a wide conformation despite the clamp domain adopting a closed configuration. The Pol I stalk—containing the A43/A14 subunits—is tightly associated with the main body of Pol I, suggesting that Pol I and Pol II rely on partially overlapping but likely distinct conformational rearrangements to alter the conformation of the DNA-binding cleft [4] , [5] . Structure of the Rpo3/Rpo11 heterodimer Rpo3 and Rpo11 of Tko RNAP form a two-fold pseudosymmetrical heterodimer comprising full-length Rpo11 and domain 1 of Rpo3 that is flanked by the two additional domains of Rpo3 ( Fig. 2b , left), and this domain organization is well conserved in the archaeal–eukaryotic RNAP family (AC40/AC19 in Pol I/Pol III, Rpb3/Rpb11 in Pol II; Supplementary Fig. 3a ) [4] , [5] , [18] , [22] . However, the architectures of domains 2 and 3 are distinct in each Rpo3, Rpb3 and AC40 subunits. Comparisons of crenarchaeal and euryarchaeal Rpo3 reveal no structural homology within domain 3. A ferredoxin-like 4Fe-4S cluster-binding domain containing the 3Fe-4S cluster plus a disulfide bond dominates the Sso Rpo3 folding, whereas domain 3 of Tko Rpo3 adopts a structure containing a pair of α-helixes covered by four β-strands. Substantial differences within domain 2 are also evident, with domain 2 of Sso Rpb3 containing two pairs of disulfide bonds, whereas no Cys residues are present in Tko Rpo3. Similarly, disparate folds of domains 2 and 3 are present in the AC40 and Rpb3. The Rpo3/Rpo11 heterodimer is on the opposite surface of the DNA-binding channel, and as such these different domains of Rpo3 are surface-exposed and in position to provide unique and specific interfaces for transcription factors binding near upstream DNA in the PIC. Consistently, in the Pol II-dependent transcription, domain 2 of Rpb3 is one of the binding targets of the Mediator [23] (further description in Discussion). Structural differences between Tko RNAP and yeast Pol II The overall sequence identity of Tko RNAP and yeast Saccharomyces cerevisiae Pol II is only 39% ( Supplementary Table 1 ), complicating simple amino-acid sequence alignments. The strong conservation of the overall fold of these RNAP structures permitted structure-guided sequence alignments ( Supplementary Figs 4 and 5 ) that provided precise comparisons of amino-acid sequences of these RNAPs. These alignments identified regions where insertions—defined as ≥4 residues—were retained in each RNAP. Tko RNAP has four unique insertions compared with Pol II, whereas yeast Pol II contains 30 distinct insertions compared with Tko RNAP ( Fig. 4 and Supplementary Fig. 4 ). Most Pol II insertions are on the surface of Pol II and 18 insertions are fully or partially disordered in the yeast Pol II crystal structure [24] . In all, 27 of the 30 Pol II insertions are conserved in human Pol II, suggesting that these insertions play fundamental roles in the Pol II-dependent transcription ( Fig. 4 and Supplementary Table 3 ). We also compared these 30 insertions with the crystal structure of Pol I (refs 4 , 5 ) and a homology model of Pol III (ref. 25 ) and identified that 13 insertions are unique in the Pol II structure (Pol II-specific insertions; Supplementary Fig. 6 and Supplementary Movie 3 ). 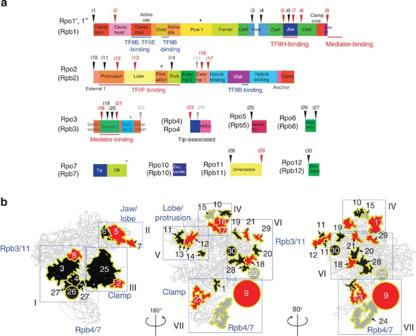Figure 4: Structural differences between theTkoRNAP and yeast Pol II. (a) Schematic diagrams of domains and domain-like regions of theTkoRNAP based on the Pol II nomenclature. Inverted triangles indicate positions of 30 insertions found in yeast Pol II compared withTkoRNAP (black, insertions in eukaryotic RNAPs; red, Pol II-specific insertions; grey, unique in yeast Pol II). The binding sites of TFIIB, TFIIE, TFIIF, TFIIH and Mediator are indicated. Asterisks indicate positions of four insertions found in theTkoRNAP subunits. (b) The structure of yeast Pol II and the three-dimensional representation of the 30 insertions ina. Insertions are depicted by plain surfaces with yellow boundaries (colours same as ina). Circles show approximate locations of disordered insertions at N- or C termini of subunits (for example, Pol II CTD) and their diameters represent their approximate lengths. Seven groups of insertions (I–VII) are indicated in blue rectangles. Figure 4: Structural differences between the Tko RNAP and yeast Pol II. ( a ) Schematic diagrams of domains and domain-like regions of the Tko RNAP based on the Pol II nomenclature. Inverted triangles indicate positions of 30 insertions found in yeast Pol II compared with Tko RNAP (black, insertions in eukaryotic RNAPs; red, Pol II-specific insertions; grey, unique in yeast Pol II). The binding sites of TFIIB, TFIIE, TFIIF, TFIIH and Mediator are indicated. Asterisks indicate positions of four insertions found in the Tko RNAP subunits. ( b ) The structure of yeast Pol II and the three-dimensional representation of the 30 insertions in a . Insertions are depicted by plain surfaces with yellow boundaries (colours same as in a ). Circles show approximate locations of disordered insertions at N- or C termini of subunits (for example, Pol II CTD) and their diameters represent their approximate lengths. Seven groups of insertions (I–VII) are indicated in blue rectangles. Full size image Notably, Pol II-specific insertions map precisely to the previously established binding sites of transcription factors unique to the Pol II transcription system (for example, TFIIF, TFIIH and Mediator) [23] , [26] , [27] , [28] and do not map to the binding sites of common GTFs shared among the archaeal RNAP and Pol II (for example, TFB/TFIIB and TFE/TFIIE; Figs 4a and 5 and Supplementary Movie 3 ). This disparity indicates that the insertions retained in extant Pol II might have been adopted as unique binding surfaces for specific transcription factors in the Pol II transcription system. For clarity, the 30 insertions (i1–i30) were separated into seven groups (Groups I–VII; Fig. 4b and Table 1 ) for further structure–function analysis based on their clustered locations and interactions with TFIIF, TFIIH and Mediator (in Discussion). 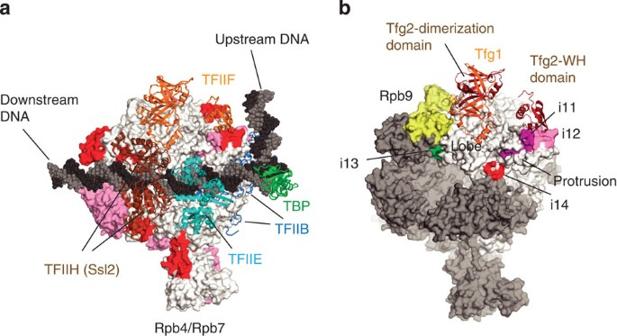Figure 5: The PIC model of Pol II. (a) Pol II, GTFs and DNA are depicted by surface, cartoon and cpk models, respectively. Insertions specific and nonspecific to Pol II are indicated in red and pink, respectively. Each GTF is denoted by a unique colour and labelled. (b) The Pol II and TFIIF interactions in the PIC. Pol II and TFIIF are depicted by surface and cartoon models, respectively. Rpb2 and Rpb9 are in white and yellow, respectively, and all other subunits are in grey. Subunits and domains of TFIIF are labelled. Four insertions participated in the TFIIF binding are indicated. This PIC model is adapted from ref.37. Figure 5: The PIC model of Pol II. ( a ) Pol II, GTFs and DNA are depicted by surface, cartoon and cpk models, respectively. Insertions specific and nonspecific to Pol II are indicated in red and pink, respectively. Each GTF is denoted by a unique colour and labelled. ( b ) The Pol II and TFIIF interactions in the PIC. Pol II and TFIIF are depicted by surface and cartoon models, respectively. Rpb2 and Rpb9 are in white and yellow, respectively, and all other subunits are in grey. Subunits and domains of TFIIF are labelled. Four insertions participated in the TFIIF binding are indicated. This PIC model is adapted from ref. 37 . Full size image Table 1 Pol II insertions (I–VII) and their interactions with GTFs and Mediator. Full size table Here we report the first crystal structure of euryarchaeal RNAP from Tko . The open-clamp conformation adopted by Tko RNAP is coupled with a rotational and swinging movement of the stalk. These coordinated movements resolve a long-standing question of how potential steric clashes between the clamp and the stalk of archaeal RNAP and Pol II can be reconciled. The Tko RNAP structure gives a structural basis for the understanding of the clamp-conformation changes of archaeal RNAP and Pol II during the transcription cycle [21] , [29] , [30] . The clamp is a conserved mobile domain in all multisubunit cellular RNAPs, and the conformation changes of the clamp are the key structural features throughout the transcription cycle including transcription initiation, transition to a stable elongation complex, and transcription pausing and termination. The stalk is a unique structure of archaeal–eukaryotic RNAPs, and it is located near the clamp and the RNA exit channel. The stalk also serves as a binding platform for GTFs of archaeal RNAP and Pol II (refs 31 , 32 ). A nascent RNA emerging from the active site of archaeal RNAP/Pol II also interacts with the stalk [33] , [34] . The coupled conformation change of the stalk with the clamp in archaeal RNAP and Pol II suggests that the stalk may be used to control the clamp conformation as a leverage-like structure. The binding of a nascent RNA to the stalk of archaeal RNAP has been shown to increase the processivity of transcription in vitro [34] . The interaction between a nascent RNA and the stalk may stabilize the closed-clamp state and this provides a plausible explanation for the enhancement of transcription processivity ( Fig. 6a ). On the other hand, TFE of archaeal system and TFIIEα of the Pol II system are known to interact with the base of the stalk and the tip of the clamp in PIC [21] , [26] , [35] , and it has been observed that the binding of TFIIE stabilizes the open-clamp conformation in human PIC [21] . The binding of TFE or TFIIEα on the tip of the clamp and base of the stalk may stabilize the open-clamp conformation with the stalk as a leverage-like role ( Fig. 6b ). 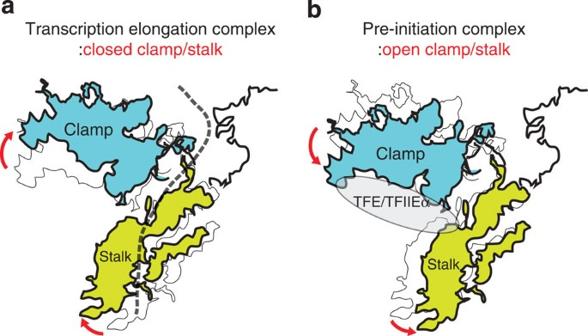Figure 6: Model of clamp-conformation control through the stalk. (a) A nascent RNA, depicted as a dashed line, may stabilize the closed conformation of the clamp in the transcription elongation complex by the interaction with the stalk. (b) Binding of TFE/TFIIEα, shown as a grey ellipse, on the clamp and stalk may stabilize the open conformation of the clamp and stalk in the PIC. Figure 6: Model of clamp-conformation control through the stalk. ( a ) A nascent RNA, depicted as a dashed line, may stabilize the closed conformation of the clamp in the transcription elongation complex by the interaction with the stalk. ( b ) Binding of TFE/TFIIEα, shown as a grey ellipse, on the clamp and stalk may stabilize the open conformation of the clamp and stalk in the PIC. Full size image Structure-guided sequence alignments between Tko RNAP and yeast Pol II revealed ~30 Pol II insertions ( Fig. 4b and Table 1 ), and there is a correlation between their locations and the proposed binding surfaces for the Pol II-specific GTFs (TFIIF and TFIIH) and Mediator. The molecular details of such interactions are largely unknown, and it is illustrative to highlight some of the known and predicted interactions that occur between Pol II-specific GTFs and these grouped insertions. Such structure-guided analyses may establish targets for more specific biochemical assays probing the molecular mechanisms of Pol II-specific GTFs during transcription initiation and early elongation. TFIIF consists of two conserved subunits, Tfg1 and Tfg2 (ref. 6 ), and several domains of Tfg2 were biochemically mapped to the Pol II lobe and protrusion domains, respectively [26] , [36] ( Fig. 5b ). Group V insertions are located on the lobe, protrusion and fork domains, and may participate in the binding of the Tfg2 subunit of TFIIF to Pol II ( Figs 5b and 7a , Table 1 and Supplementary Movie 3 ) [26] , [37] . It should be noted that the amino-acid residues on Pol II that interact with TFIIF are not conserved in Pol I and Pol III ( Supplementary Fig. 7a ). 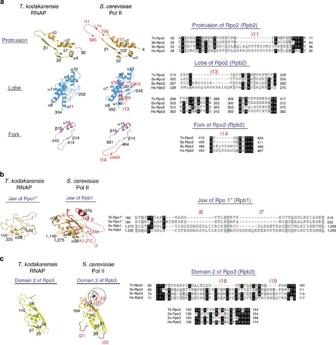Figure 7: Structure and sequence comparisons ofTkoRNAP and yeast Pol II around binding sites of the Pol II-specific GTFs/Mediator. Structures of Pol II around the binding sites of TFIIF (a), TFIIH (b) and Mediator (c) and their counterparts in theTkoRNAP structure are shown. Insertions are coloured and indicated in red, and disordered regions are depicted as dashed lines. Amino-acid sequence alignments around these regions are shown on their right (Tk,Tko; Ss,Sso; Sc,Sce; Hs,Homo sapiens). Amino-acid residues crosslinked to TFIIF (a) and TFIIH (b) are indicated in red. Cys92 and Ala159 of Rpb3, which interact directly with the Mediator, are indicated in red and the positions of i18 are indicated by a blue arrow onTkoRNAP and a blue circle on Pol II (c). Figure 7: Structure and sequence comparisons of Tko RNAP and yeast Pol II around binding sites of the Pol II-specific GTFs/Mediator. Structures of Pol II around the binding sites of TFIIF ( a ), TFIIH ( b ) and Mediator ( c ) and their counterparts in the Tko RNAP structure are shown. Insertions are coloured and indicated in red, and disordered regions are depicted as dashed lines. Amino-acid sequence alignments around these regions are shown on their right (Tk, Tko ; Ss, Sso ; Sc, Sce ; Hs, Homo sapiens ). Amino-acid residues crosslinked to TFIIF ( a ) and TFIIH ( b ) are indicated in red. Cys92 and Ala159 of Rpb3, which interact directly with the Mediator, are indicated in red and the positions of i18 are indicated by a blue arrow on Tko RNAP and a blue circle on Pol II ( c ). Full size image TFIIH was proposed to bind to a surface connecting the jaw, clamp and stalk domains of Pol II; however, the molecular details of the interface remain unknown [21] , [28] , [37] . The Pol II-specific insertions i2, i5, i7 and i23 bridge the jaw, clamp and stalk domains of Pol II, suggesting that these insertions might be involved in direct interactions with TFIIH ( Fig. 8a ). The density connecting the stalk and TFIIH in the cryo-EM study of human PICs corresponds to i23 (ref. 21 ), and i5 and i7 are positioned to potentially interact with the C-terminal domain (CTD) of Ssl2 (refs 28 , 37 ; Fig. 7b ). Insertion 2 in the clamp head domain may represent an addition contact site as suggested by a cryo-EM/crosslinking study of yeast PIC [28] . 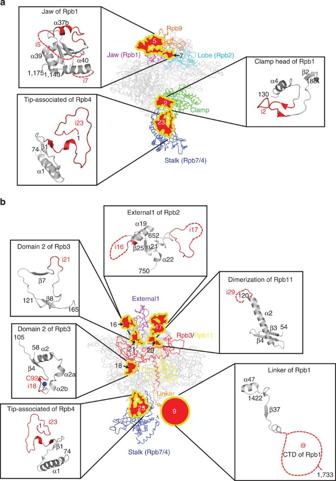Figure 8: Pol II-specific insertions and TFIIH- and Mediator-binding interfaces on Pol II. (a) Pol II-specific insertions on the Pol II backbone model on the TFIIH-binding interface. (b) Pol II-specific insertions on the Mediator-binding interface. In both panels, insertions are shown as red plain surfaces with yellow-green boundaries on the Pol II backbone model, and the key subunits and domains are indicated. Magnified views of these insertions are shown in boxes. Figure 8: Pol II-specific insertions and TFIIH- and Mediator-binding interfaces on Pol II. ( a ) Pol II-specific insertions on the Pol II backbone model on the TFIIH-binding interface. ( b ) Pol II-specific insertions on the Mediator-binding interface. In both panels, insertions are shown as red plain surfaces with yellow-green boundaries on the Pol II backbone model, and the key subunits and domains are indicated. Magnified views of these insertions are shown in boxes. Full size image The cryo-EM structures of Pol II in complex with Mediator suggested extensive interactions between Pol II and Mediator [38] , [39] and no fewer than seven Pol II subunits (Rpb1, Rpb2, Rpb3, Rpb4, Rpb6, Rpb7 and Rpb11) were proposed to be involved in this interaction. Although a massive Pol II–Mediator interaction surface is likely, the molecular details facilitating such interactions are currently limited to a few surfaces including the structurally unresolved CTD of Rpb1 (ref. 27 ) and Cys92/Ala159 in domain 2 of Rpb3 (ref. 23 ). Our structural analysis shows that Cys92 is located within Pol II-specific insertion i18 and participates in coordinating a zinc ion with three other cysteines to form the Zn loop of Rbp3 ( Fig. 7c ). This structure is conserved in Pol II from yeast to humans but is not conserved in the AC40 counterpart of Pol I/Pol III ( Supplementary Fig. 7b ). As noted earlier, the domain 2 structures of the Rpb3 homologues in Pol I/Pol III (AC40 subunit) or archaeal RNAP (Rpo3 subunit) share no structural similarity ( Supplementary Fig. 3a ) indicating that unique surface-exposed insertion regions may represent the binding sites for Pol II-specific regulatory complexes. Pol II-specific insertions in Group IV, VI and VII insertions locate to the opposite side of the enzyme from the DNA-binding cleft ( Fig. 8b and Supplementary Movie 3 ) containing the well-characterized Mediator-binding sites including the CTD (i9) and the Zn loop of Rpb3 (i18). The insertions elucidated from these structural analyses provide logical positions to further investigate the Pol II–Mediator interaction. Purification and crystallization of the Tko Rpo3/Rpo11 A polycistronic plasmid (pET21a-Rpo3-Rpo11) was generated to simultaneously overexpress the genes encoding Tko Rpo3 and Rpo11. Escherichia coli BL21-CodonPlus(DE3)-RIPL (Stratagene) cells were transformed with pET21a-Rpo3-Rpo11, and transformants were grown in LB media supplemented with 100 μg ml −1 of ampicillin at 37 °C to an OD600 of ~0.8 before the addition of isopropyl-β-D-thiogalactoside to 0.5 mM final to induce expression. Cells were harvested 5 h post induction, suspended in lysis buffer (20 mM Tris–HCl (pH 8.0), 50 mM KCl, 10 mM β-mercaptoethanol, 5 % glycerol and protease inhibitor cocktail (Roche)) and lysed with sonication. The Rpo3/Rpo11 complex was purified from the lysate by heat treatment at 65 °C for 30 min, followed by passage and fractionation of the cleared supernatant through two separate chromatographic columns (Q-sepharose and Superdex-75 gel filtration column chromatography, GE Healthcare). A selenomethionine (SeMet)-substituted Rpo3/Rpo11 complex was prepared by suppression of methionine biosynthesis [40] during culture growth, followed by an identical purification scheme as for the native complex. Both native and SeMet-labelled Rpo3/Rpo11 were concentrated to 10 mg ml −1 with buffer (10 mM Tris–HCl (pH 8), 50 mM NaCl, 1 mM EDTA and 2 mM dithiothreitol (DTT)) for crystallization. Microbatch crystallization, mixing protein and crystallization solutions, was performed under a thin layer of paraffin oil at 4 °C against a reservoir containing 0.1 M CAPS (pH 10), 0.1 M ammonium dihydrogen phosphate and 34% (w/v) PEG4000. Crystals reached their full size (0.15 × 0.10 × 0.10 mm, diamond shape) within 2 weeks. Cryoprotection of the crystal was achieved by stepwise transfer to a crystallization solution containing 45% (w/v) PEG4000, and the crystals were flash-frozen using liquid nitrogen. Structure determination of Tko Rpo3/Rpo11 The data sets Native and SeMet were collected at the National Synchrotron Light Source (Brookhaven National Laboratory, Upton, NY, USA) Beamline X25 at 100 K. All data sets were processed by HKL2000 (ref. 41 ). For SeMet multiwavelength anomalous dispersion phasing, 14 Se atom positions were identified by the programme SnB [42] and the initial phase was calculated by SOLVE [43] followed by automated model building by RESOLVE [44] . The partial model was refined using the native protein data set and the final model was built manually using O [45] and refined using CNS [46] at 1.6 Å resolution ( Supplementary Table 2 ). The crystal belongs to the primitive orthorhombic space group and contains two structurally identical Rpo3/Rpo11 complexes in each asymmetric unit. Ninety-eight per cent of the residues fall in favoured regions of the Ramachandran plot and none of them is in disallowed regions. Purification and crystallization of the Tko Rpo4/Rpo7 A polycistronic plasmid (pET21a-Rpo4-Rpo7) was generated to simultaneously overexpress the genes encoding Tko Rpo7 and Rpo4. Rpo4/Rpo7 was expressed and purified as described for the preparation of Tko Rpo3/Rpo11. The purified Rpo4/Rpo7 complex was concentrated to 30 mg ml −1 with buffer (10 mM Tris–HCl (pH 8), 50 mM NaCl, 0.1 mM EDTA and 1 mM DTT) for crystallization. Crystals were obtained using hanging-drop vapour diffusion by mixing equal volumes of Rpo4/Rpo7 and crystallization solution (0.1 M NaAcetate (pH 5.0) and 30% glycerol) and incubating at 22 °C over the same crystallization solution. Crystals were directly frozen using liquid nitrogen. Structure determination of Tko Rpo4/Rpo7 X-ray diffraction data were collected at the X-ray core facility at Pennsylvania State University at 100 K and the data set was processed by HKL2000 (ref. 41 ). The structure of the Sso Rpo4/Rpo7 complex from the complete Sso RNAP [18] was used as a search model for molecular replacement. Positional refinement was performed using Refmac5 (ref. 47 ) and Phenix [48] and the resulting map was used for building the final model manually by Coot [49] . The final structure was refined at 2.3 Å resolution ( Supplementary Table 2 ). The crystal belongs to the primitive orthorhombic and contains one Rpo4/Rpo7 in an asymmetric unit. Ninety-four per cent of the residues fall in favoured regions of the Ramachandran plot and 2% of them are in disallowed regions. Purification and preparation of Tko RNAP Tko Δ Rpo4 strain, KUWLFB [16] , was grown under anaerobic conditions at 75 °C in nutrient-rich media (ASW-YT) containing 0.5% yeast extract (Y) and 0.5% trypton (T) in artificial seawater [16] . Two litres seed culture were inoculated into 200 l batch cultures, and cells were grown for ~20 h until reaching mid-log phase. For RNAP purification, 50 g of cells were suspended in 200 ml lysis buffer (10 mM Tris–HCl (pH 8.0), 500 mM KCl, 10% glycerol, 10 mM imidazole, 10 μM ZnCl 2 , 5 mM 2-mercaptoethanol, 0.3 μM leupeptin, 1 μM pepstatin, 1.5 mM benzamidine hydrochloride and 0.5 mM phenylmethyl sulphonyl fluoride) and lysed by an Emulsiflex C3 homogenizer (Avestin Inc.) at 20,000 p.s.i. After centrifugation (27,000 g for 1 h), the supernatant was loaded to 2 × 5 ml tandemly linked Ni-NTA affinity columns (Qiagen) equilibrated with the lysis buffer and washed with the same buffer containing 20 mM imidazole. Proteins were eluted with the lysis buffer containing 200 mM imidazole and precipitated by ammonium sulfate (final 80% saturation). The pellet was suspended in TGED buffer (20 mM Tris–HCl (pH 8.0), 10% glycerol, 0.5 mM EDTA and 5 mM DTT) until its conductivity was below 10 S m −1 and RNAP was further purified by binding and elution from a 5-ml HiTrap Q HP (GE Healthcare) column following a linear KCl gradient from 0.1 to 0.4 M. SDS–polyacrylamide gel electrophoresis analysis of fractions resultant from HiTrap Q chromatography revealed a mixture of RNAP complexes lacking Rpo4/Rpo7 and RNAP complexes lacking Rpo4. To reconstitute RNAP containing all subunits, both RNAP pools from HiTrap Q were mixed with recombinant Rpo4/Rpo7 and Rpo4 at a ratio of 1:4:1 (RNAP:Rpo4/Rpo7:Rpo4) for 1 h at 20 °C and were further purified by successive passage and elution from 5 ml HiTrap Heparin, 8 ml MonoQ and Superdex200 columns (GE healthcare). Approximately 5 mg of 11-subunit Tko RNAP was obtained from each 50-g preparation. Crystallization and structure determination of Tko RNAP Tko RNAP was concentrated to 10 mg ml −1 in buffer (10 mM Tris-HCl (pH 8.0), 200 mM KCl, 5 % glycerol, 10 μM ZnCl 2 , 5 mM DTT and 0.1 mM EDTA), and the crystals were grown by hanging-drop vapour diffusion by mixing 1.2 μl of RNAP and 1 μl of reservoir solution (0.1 M imidazole (pH 8.0), 0.2 M CaCl 2 , 0.2 M NaNO 3 and 12% PEG8000) at 22 °C. The crystals appeared in 3 days and grew to full size (0.1 × 0.05 × 0.3 mm) in 2 weeks. For cryocrystallography, the crystals were transferred stepwise over a period of 5 min to 20% ethylene glycol in 5% increments and flash-frozen in liquid N 2 . The crystals belong to the space group P2 1 2 1 2 1 and contain two Tko RNAPs per asymmetric unit. Diffraction data were collected at the Macromolecular Diffraction line at the Cornell University High Energy Synchrotron Source (MacCHESS) F1 beamline (Cornell University, Ithaca, NY, USA) at 100 Kn and data were processed by HKL2000 (ref. 41 ). The structure of Tko RNAP was determined by molecular replacement using AutoMR in Phenix [48] . A search model for the molecular replacement was prepared from the Sso RNAP structure (PDB: 3 HKZ) [1] with the following modifications: (i) Tko Rpo3/Rpo11 and Rpo4/Rpo7 subcomplexes replaced their counterparts in Sso RNAP and (ii) RpoG and Rpo13 were removed from the Sso coordinates. In the course of the structure determination of Tko RNAP, a substantial difference was noted in the position of the clamp domain compared with the clamp position determined for Sso RNAP. Therefore, we removed the clamp domain of Sso RNAP from the search model. After rigid body refinement and deformable elastic network (DEN) refinement using Crystallography & NMR System (CNS) [50] , the electron-density map was interpreted and traced with Coot [49] . The crystal structure of clamp domain of Pfu RNAP (PDB ID 3QQC, chain A) had been determined [51] , and we therefore fitted this structure manually into the electron-density map corresponding to the region specified for the Tko RNAP clamp domain. Further refinement was performed using Phenix [48] with noncrystallographic symmetry and secondary structure restraints, and the resulting model was manually rebuilt with Coot [49] . The final position and orientation of the clamp domain of Tko RNAP were confirmed by the locations of Zn ions. Ninety-five per cent of the residues fall in favoured regions of the Ramachandran plot and five per cent of them are in the disallowed regions. Phylogenetic analysis Amino-acid sequences of the largest subunits of RNAPs from bacteria, archaea and eukaryote were aligned by Muscle with default parameters, and a phylogenetic tree was constructed using the Molecular Evolutionary Genetics Analysis (MEGA6) [52] with maximum-likelihood method using Jones–Taylor–Thormton model, uniform rate and bootstrap replication of 500 times. Accession codes: Coordinates and structure factors have been deposited in the Protein Data Bank with accession codes: 4QIW , Tko RNAP; 4QJV , Rpo3/Rpo11; 4QJF, Rpo4/Rpo7. How to cite this article: Jun, S.-H. et al. The X-ray crystal structure of the euryarchaeal RNA polymerase in an open-clamp configuration. Nat. Commun. 5:5132 doi: 10.1038/ncomms6132 (2014).